Superionic glass-ceramic electrolytes for room-temperature rechargeable sodium batteries Innovative rechargeable batteries that can effectively store renewable energy, such as solar and wind power, urgently need to be developed to reduce greenhouse gas emissions. All-solid-state batteries with inorganic solid electrolytes and electrodes are promising power sources for a wide range of applications because of their safety, long-cycle lives and versatile geometries. Rechargeable sodium batteries are more suitable than lithium-ion batteries, because they use abundant and ubiquitous sodium sources. Solid electrolytes are critical for realizing all-solid-state sodium batteries. Here we show that stabilization of a high-temperature phase by crystallization from the glassy state dramatically enhances the Na + ion conductivity. An ambient temperature conductivity of over 10 −4 S cm −1 was obtained in a glass-ceramic electrolyte, in which a cubic Na 3 PS 4 crystal with superionic conductivity was first realized. All-solid-state sodium batteries, with a powder-compressed Na 3 PS 4 electrolyte, functioned as a rechargeable battery at room temperature. Sodium-ion rechargeable batteries, using abundant sodium sources, are suitable for use in distributed power systems that store renewable energy at individual houses [1] , [2] , [3] , [4] . Currently, sodium−sulphur (NAS) batteries [5] are used for large-scale storage, because they have high energy densities of up to 760 Wh kg −1 . However, NAS batteries need to be operated at temperatures up to 300 °C to use liquid-state sulphur-positive electrodes and sodium-negative electrodes and to enhance the conductivity of β-alumina solid electrolyte, a well-known Na + ion conductor. From a safety viewpoint, NAS batteries that operate at room temperature are strongly desirable as they would be a suitable distributed storage for individual houses. All-solid-state batteries are the safest batteries, because they do not suffer from leakage, volatilization, or flammability, as they employ solid inorganic electrolytes rather than liquid organic electrolytes [6] , [7] , [8] . To realize solid-state batteries that operate at ambient and moderate temperatures, superior solid electrolytes that have high Na + ion conductivities at room temperature and close contact with electrode active materials are indispensable. Moreover, a drastic reduction in the interparticle resistance of electrolytes without high-temperature sintering is highly significant, because this is critical for developing large-scale solid-state batteries. However, no highly conductive electrolytes suitable for room-temperature operation of batteries have been found [9] , [10] , [11] , [12] , [13] , [14] , [15] . We have studied Li + ion conducting electrolytes and found that solid sulphide electrolytes made from the system Li 2 S–P 2 S 5 have a high conductivity and a wide electrochemical window [16] , [17] , making them suitable for all-solid-state lithium secondary batteries that have excellent cycling and rate performances [18] , [19] , [20] , [21] . In this study, we developed a sulphide glass-ceramic electrolyte by crystallization of high-temperature cubic Na 3 PS 4 phase from the glassy state. The prepared electrolyte showed a sodium-ion conductivity of 2×10 −4 S cm −1 at room temperature. This high conductivity was achieved by stabilization of cubic Na 3 PS 4 and large reduction of grain-boundaries in a glass-ceramic pellet. A room-temperature operation of all-solid-state rechargeable sodium batteries with a powder-compressed glass-ceramic electrolyte was first realized and this achievement is the first step toward realizing all-solid-state NAS batteries. Crystallization of Na 3 PS 4 glass electrolytes Ortho-thiophosphate Na 3 PS 4 glass was prepared by a mechanochemical technique using a planetary ball mill; the synthesized sample exhibited a halo pattern in its X-ray diffraction (XRD) pattern ( Fig. 1a ) and a glass transition at 180 °C in differential thermal analysis (DTA, Fig. 1d ). A Raman spectrum of the glass ( Fig. 1e ) revealed that the glass had a single band at 420 cm −1 , which is attributable to the ortho-thiophosphate ion (PS 4 3− ) (ref. 22 ). This implies that the glass had the nominal composition. 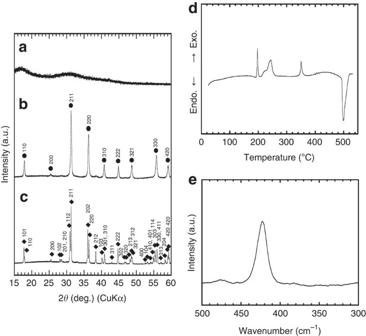Figure 1: Characterization of the Na3PS4glass and glass-ceramic electrolytes. (a,b,c) XRD patterns of the Na3PS4glass (a), glass-ceramic sample heated at 270 °C (b), and glass-ceramic sample heated at 420° C (c). Closed circles and diamonds, respectively, denote the diffraction peaks attributable to the cubic Na3PS4phase and the tetragonal Na3PS4phase (JCPDS #081-1472). (d) DTA curve of the Na3PS4glass. (e) Raman spectrum of the Na3PS4glass. Figure 1: Characterization of the Na 3 PS 4 glass and glass-ceramic electrolytes. ( a , b , c ) XRD patterns of the Na 3 PS 4 glass ( a ), glass-ceramic sample heated at 270 °C ( b ), and glass-ceramic sample heated at 420° C ( c ). Closed circles and diamonds, respectively, denote the diffraction peaks attributable to the cubic Na 3 PS 4 phase and the tetragonal Na 3 PS 4 phase (JCPDS #081-1472). ( d ) DTA curve of the Na 3 PS 4 glass. ( e ) Raman spectrum of the Na 3 PS 4 glass. Full size image As shown in Fig. 1b , a crystalline phase was precipitated after heating the Na 3 PS 4 glass at 270 °C, which is above the first crystallization temperature determined by DTA. The XRD pattern of the glass-ceramic (that is, crystallized glass) was indexed by a cubic phase based on a tetragonal phase of Na 3 PS 4 (JCPDS #081-1472). Cubic Na 3 PS 4 is considered to be a high-temperature phase of tetragonal Na 3 PS 4 (ref. 12 ), but the cubic phase of Na 3 PS 4 has not been reported previously. The glass-ceramic obtained by heating at a higher temperature of 420 °C had a different XRD pattern that is attributable to the low-temperature phase of tetragonal Na 3 PS 4 (ref. 12 ) ( Fig. 1c ). Electrical conductivity of Na 3 PS 4 solid electrolytes A powder-compressed pellet of the Na 3 PS 4 glass and the glass-ceramic pellet prepared at 270 °C with carbon electrodes on both surfaces were evaluated by alternating current impedance measurements. 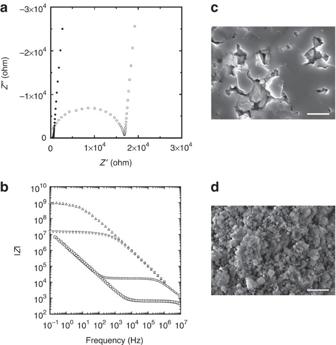Figure 2: Impedance and morphology of the Na3PS4glass, the Na3PS4glass-ceramic and β-alumina electrolytes. (a) Impedance plots at 25 °C of a powder-compressed pellet of the Na3PS4glass (open circle) and the glass-ceramic pellet prepared at 270 °C (closed circle). (b) Bode plots of the pellets of the Na3PS4glass (open circle, at 25 °C) and the Na3PS4glass-ceramic (open square, at 25 °C), and the β-alumina (open triangle (at 70 °C) and open reverse-triangle (at 120 °C)). (c,d) Cross-sectional SEM images of the Na3PS4glass-ceramic pellet (c) and the β-alumina pellet (d). Scale bar, 5 μm. Figure 2a shows impedance plots of the pellets. The impedance plots of the glass pellet exhibit a semicircle and a spike in the low-frequency region, suggesting that the glass behaves as a typical ionic conductor. The total conductivity, which includes the bulk-grain and grain-boundary resistances, was determined from the cross-sectional resistance between the semicircle and the spike on the x axis. In contrast, impedance plots of the pellet of the glass-ceramic with the cubic Na 3 PS 4 phase exhibits only a spike and the resistance of the pellet decreases by a factor of 30 on crystallization. Figure 2: Impedance and morphology of the Na 3 PS 4 glass, the Na 3 PS 4 glass-ceramic and β-alumina electrolytes. ( a ) Impedance plots at 25 °C of a powder-compressed pellet of the Na 3 PS 4 glass (open circle) and the glass-ceramic pellet prepared at 270 °C (closed circle). ( b ) Bode plots of the pellets of the Na 3 PS 4 glass (open circle, at 25 °C) and the Na 3 PS 4 glass-ceramic (open square, at 25 °C), and the β-alumina (open triangle (at 70 °C) and open reverse-triangle (at 120 °C)). ( c , d ) Cross-sectional SEM images of the Na 3 PS 4 glass-ceramic pellet ( c ) and the β-alumina pellet ( d ). Scale bar, 5 μm. Full size image The conductivities of the Na 3 PS 4 glass and glass-ceramic were compared with the conductivity of β-alumina as a typical Na + ion conductor. A pellet of β-alumina was prepared by cold-pressing its powders, which had been sufficiently pulverized, and its impedance was measured as a function of frequency. Figure 2b shows Bode plots of the electrolyte pellets of the Na 3 PS 4 glass (25 °C), the glass-ceramic (25 °C), and β-alumina (70 and 120 °C). (The data for the glass and glass-ceramic are the same as those shown in Fig. 2a ). The absolute values of impedance | Z | as a function of frequency of β-alumina behave completely differently from those of the Na 3 PS 4 glass and glass-ceramic. The glass-ceramic has smaller impedance than β-alumina in the high-frequency range from 10 4 to 10 7 Hz, whereas the impedance of β-alumina at 70 °C is six orders of magnitude larger than that of glass-ceramic at low frequencies in the range 0.1 to 10 Hz. This is clear evidence that the Na 3 PS 4 glass-ceramic pellet possesses a higher ionic motion than the β-alumina pellet. Cross-section of the pellets was analysed by scanning electron microscope (SEM). Grain-boundaries among particles are clearly observed in the β-alumina pellet ( Fig. 2d ), whereas intimate contacts among particles are achieved in the Na 3 PS 4 glass-ceramic pellet ( Fig. 2c ). The difference in microstructure affects the total conductivity (especially conductivity at grain-boundary) of the pellets. 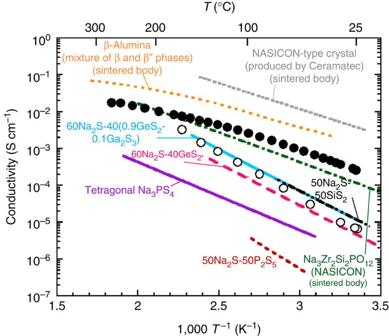Figure 3: Conductivity of the Na3PS4glass and glass-ceramic electrolytes. Temperature dependences of the conductivities of the Na3PS4glass (open circles) and the glass-ceramic prepared at 270 °C (solid circles). Conductivities of several Na+ion conductors reported so far are also shown as a comparison. Figure 3 shows the electrical conductivities of Na 3 PS 4 glass, glass-ceramic electrolytes, and typical inorganic solid electrolytes [9] , [10] , [11] , [12] , [13] , [14] , [15] that have Na + ion conductivities. All the conductivities in this figure were determined from the total resistance, which includes both bulk-grain and grain-boundary components. The Na 3 PS 4 glass pellet (open circles) has a conductivity of 6×10 −6 S cm −1 at room temperature and an activation energy for conduction of 47 kJ mol −1 ; it has similar conductivity properties to those of sulphide glasses in systems such as Na 2 S–SiS 2 and Na 2 S–GeS 2 (refs 9 , 10 , 11 . On the other hand, the glass-ceramic with cubic Na 3 PS 4 (closed circles) has a conductivity of 2×10 −4 S cm −1 at room temperature and an activation energy of 27 kJ mol −1 . The presence of cubic Na 3 PS 4 is responsible for the large increase in the conductivity of the glass-ceramic electrolyte because tetragonal Na 3 PS 4 , which is the low-temperature phase, has a conductivity of 1×10 −6 S cm −1 at room temperature [12] . The Na 3 PS 4 glass-ceramic electrolyte has a higher conductivity than sulphide glasses [9] , [10] , [11] and a Na 3 Zr 2 Si 2 PO 12 NASICON crystal [14] . Several sintered electrolytes such as β-alumina (consisting of β and β″ phases) [13] and a NASICON-type crystal (produced by Ceramatec) [15] have a higher conductivity of 10 −3 S cm −1 at room temperature; sintering at a high temperature of 1,800 °C is needed to reduce the grain-boundary resistance for β-alumina [13] . Although the conductivity of the Na 3 PS 4 glass-ceramic electrolyte is one order of magnitude lower than that of sintered β-alumina and the NASICON-type crystal, the use of the sulphide glass-ceramic results in good electrode–electrolyte contact by simple cold pressing. Figure 3: Conductivity of the Na 3 PS 4 glass and glass-ceramic electrolytes. Temperature dependences of the conductivities of the Na 3 PS 4 glass (open circles) and the glass-ceramic prepared at 270 °C (solid circles). Conductivities of several Na + ion conductors reported so far are also shown as a comparison. Full size image Application to all-solid-state sodium batteries The electrochemical window of the sulphide glass-ceramic electrolyte with cubic Na 3 PS 4 was examined by performing cyclic voltammetry measurements. As shown in Fig. 4 , reversible sodium deposition and dissolution currents were observed at about 0 V versus Na + /Na, and no remarkable oxidation currents were observed up to 5 V. This suggests that the sulphide electrolyte has a wide electrochemical window of 5 V and is electrochemically stable against Na metal. 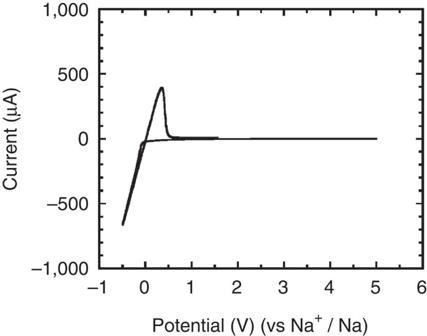Figure 4: Cyclic voltammogram of the Na3PS4glass-ceramic electrolyte. The glass-ceramic was prepared at 270 °C. A stainless-steel disk, as the working electrode, and a sodium foil, as the counter/reference electrode, were used. The potential sweep was performed with a scanning rate of 5 mV s−1at 25 °C. Figure 4: Cyclic voltammogram of the Na 3 PS 4 glass-ceramic electrolyte. The glass-ceramic was prepared at 270 °C. A stainless-steel disk, as the working electrode, and a sodium foil, as the counter/reference electrode, were used. The potential sweep was performed with a scanning rate of 5 mV s −1 at 25 °C. Full size image All-solid-state test cells were fabricated using the Na 3 PS 4 glass-ceramic solid electrolyte. A three-layered pellet of Na–Sn alloy (counter and reference electrodes)/Na 3 PS 4 (solid electrolyte)/TiS 2 (working electrode) was prepared by cold pressing at room temperature. The TiS 2 electrode was selected as a model active material in Na + ion batteries, because of its large electronic conductivity and good electrochemical performance in organic liquid electrolyte cells [23] . 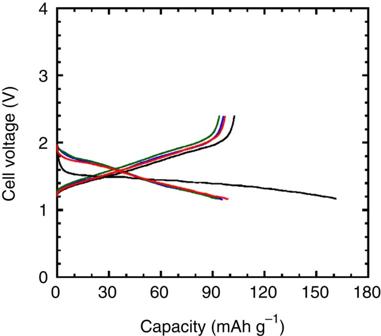Figure 5: Charge-discharge curves of the all-solid-state rechargeable sodium cell Na-Sn / Na3PS4glass-ceramic / TiS2. The black, red, blue and green lines, respectively, denote the first, second, third and tenth cycles. The cell operation was carried out at 25 °C at the current density of 0.013 mA cm−2. Figure 5 shows charge–discharge curves of the all-solid-state cell (Na–Sn/Na 3 PS 4 /TiS 2 ) at room temperature. The cell operated as a rechargeable sodium battery at room temperature. The average cell voltages from the second to tenth cycles were 1.6 V, which approximately correspond to the potential difference between the Na–Sn counter electrode (ca. 0.3 V versus Na + /Na) [24] and the TiS 2 working electrode (ca. 2.0 V versus Na + /Na) [23] . The reversible capacity of the cell was about 90 mAh per gram of TiS 2 and the cell kept the capacity for 10 cycles. This is the first case that room-temperature operation of all-solid-state rechargeable sodium batteries using inorganic electrolyte powders has been reported. Figure 5: Charge-discharge curves of the all-solid-state rechargeable sodium cell Na-Sn / Na 3 PS 4 glass-ceramic / TiS 2 . The black, red, blue and green lines, respectively, denote the first, second, third and tenth cycles. The cell operation was carried out at 25 °C at the current density of 0.013 mA cm −2 . Full size image A high conductivity of the Na 3 PS 4 glass-ceramic electrolyte is originally from the precipitation of the cubic Na 3 PS 4 phase from the glassy state. A high-temperature phase, such as α-AgI (Ag + superionic conductor) [25] , [26] or Li 7 P 3 S 11 (Li + superionic conductor) [16] , [17] , with a high ionic conductivity precipitates as the first crystal from a supercooled liquid above the glass transition temperature. This is the first time for sodium ion conductors that cubic Na 3 PS 4 has been stabilized as a high-temperature phase. The cubic Na 3 PS 4 phase was at least stable even after storage for half-a-year at room temperature in an Ar-filled glove box. A glass component does not completely vanish by crystallization, and thus the remaining glass part would have an important role in stabilizing a high-temperature phase, cubic Na 3 PS 4 . Detailed analysis of the glass component in the glass-ceramic electrolyte is now in progress. Oxide Na + ion conductors including β-alumina generally require high-temperature sintering to reduce their grain-boundary resistance; this sintering may deteriorate the electrode–electrolyte interface through undesirable side reactions. Therefore, the low grain-boundary resistance of the Na 3 PS 4 glass-ceramic pellet is highly advantageous for achieving good electrode–electrolyte contact in all-solid-state batteries. All-solid-state rechargeable sodium cells (Na–Sn/TiS 2 ) with a powder-compressed Na 3 PS 4 glass-ceramic electrolyte functioned at room temperature. Although the capacity was limited to nearly 40% of the theoretical capacity of TiS 2 , the all-solid-state cell has the potential to realize good charge–discharge reversibility. Utilization of active materials and rate performance would be enhanced by optimizing preparation technique of composite positive electrodes [27] , [28] and increasing conductivity of solid electrolytes by their structural modification [17] , [18] , [29] , which are based on our experimental results found in all-solid-state lithium secondary batteries. Work to improve the battery performance is currently in progress. The findings presented here represent the first step towards realizing practical all-solid-state Na + ion batteries that are safe and inexpensive. We have reported excellent cycle performance of all-solid-state lithium-sulphur batteries at room temperature by formation of intimate contact among sulphur, a glass-ceramic electrolyte and a conductive additive, using a ball-milling technique [30] , [31] . We thus believe that all-solid-state NAS batteries, which operate at room temperature, will be developed in the near future. Such next-generation batteries contribute to the realization of a low-carbon society by efficient use of sustainable energy. Preparation Na 3 PS 4 glass and glass-ceramic electrolytes Na 3 PS 4 glass was prepared by a mechanochemical technique using a planetary ball mill (Fritsch, Pulverisette 7). The starting materials of 75 mol% Na 2 S (Aldrich) and 25 mol% P 2 S 5 (Aldrich) were hand-ground and the mixture was then placed into a zirconia (ZrO 2 ) vessel (internal volume of 45 ml) with 500 ZrO 2 balls (4 mm in diameter). The mechanochemical reaction was performed for 20 h at a fixed rotation speed of the base disc of 510 r.p.m. to form Na 3 PS 4 glass powders. The contamination from the vessel and ball media was analysed by inductively coupled plasma atomic emission spectroscopy (ICP-AES; Seiko Instruments, SPS7800); the amount of ZrO 2 estimated from the amount of Zr in the milled Na 3 PS 4 glass was ca 0.1 wt%, and, thus, the trace amount of ZrO 2 would not affect conductivity and crystal phase of glass-ceramics. The glass powder was compressed by a conventional uniaxial cold press to prepare a pellet that was 10 mm in diameter and 1–1.5 mm thick. In the Na 3 PS 4 glass, several crystallization peaks were observed at 200–260 °C and at about 350 °C in the DTA curve ( Fig. 1d ), and different crystal phases were precipitated over those crystallization temperatures. To obtain glass-ceramics with different crystals, the glass pellets were crystallized by heating at 270 or 420 °C, in an electric furnace, for 2 h. All the processes were performed in a dry Ar atmosphere. Characterization of solid electrolytes XRD (MAC Science, M18XHF 22 -SRA) measurements of the prepared materials were performed using Cu Kα to identify the crystalline phases. Raman spectra of the glass were obtained using a Raman spectrophotometer (Jasco, NR-1000), using the 514 nm line of an Ar laser. DTA was performed by using a thermal analyser (Rigaku, Thermo Plus TG8110) at a heating rate of 10 °C min −1 . Microstructure of cross-section for the electrolyte pellets was observed by SEM (JEOL, JSM-6610A). The ionic conductivities of the pelletized samples were measured. Carbon paste was painted to form electrodes on both faces of the pellets. Two stainless-steel discs coupled with Pt wires were attached to the pellets as a current collector. Alternating current impedance measurements were performed for the obtained two-electrode cell in a dry Ar gas atmosphere, using an impedance analyser (Solartron, 1260) in the frequency range of 0.1 Hz to 8 MHz. Cyclic voltammetry measurements were conducted to investigate the electrochemical properties of the solid electrolytes. A stainless-steel disk as the working electrode and a sodium foil as the counter electrode were attached to each face of the pellet. The potential sweep was performed by using a potentiostat/galvanostat device (Hokuto Denko, HSV-100) with a scanning rate of 5 mV s −1 at room temperature. Evaluation of all-solid-state sodium batteries An all-solid-state test cell was fabricated using TiS 2 as the working electrode, Na 3 PS 4 glass-ceramic as the solid electrolyte, and a Na–Sn alloy as the counter and reference electrodes. The working electrode was a composite of TiS 2 active material and the solid electrolyte powders, because sodium ion paths to the active material are required to operate the cell. A reagent-grade TiS 2 (Kojundo Chemical Laboratory) and the Na 3 PS 4 glass-ceramic with the weight ratio of 2:3 were well-mixed using an agate mortar and pestle. The working electrode (10 mg) and the solid electrolyte (80 mg) powders were placed in a 10-mm-diameter polycarbonate tube and pressed together by applying a pressure of 360 MPa. A Na foil ( ca 90 μm) and Sn foil (15 μm), where the molar ratio of Na to Sn was almost 3, was then placed on the surface of the solid electrolyte side of the bilayer pellet and a pressure of 120 MPa was applied to the three-layered pellet. The three-layered pellet was sandwiched between two stainless-steel rods as current collectors. All the cell preparation processes were performed in a dry Ar-filled glove box. Electrochemical tests were conducted at a constant current density of 0.013 mA cm −2 (ca 0.01 C) in the voltage range from 1.17 to 2.40 V at room temperature under an Ar atmosphere using a charge–discharge measurement device (Nagano, BTS-2004). How to cite this article: Hayashi, A. et al . Superionic glass-ceramic electrolytes for room-temperature rechargeable sodium batteries. Nat. Commun. 3:856 doi: 10.1038/ncomms1843 (2012).